Probing the catalytic activity of porous graphene oxide and the origin of this behaviour Graphene oxide, a two-dimensional aromatic scaffold decorated by oxygen-containing functional groups, possesses rich chemical properties and may present a green alternative to precious metal catalysts. Graphene oxide-based carbocatalysis has recently been demonstrated for aerobic oxidative reactions. However, its widespread application is hindered by the need for high catalyst loadings. Here we report a simple chemical treatment that can create and enlarge the defects in graphene oxide and impart on it enhanced catalytic activities for the oxidative coupling of amines to imines (up to 98% yield at 5 wt% catalyst loading, under solvent-free, open-air conditions). This study examines the origin of the enhanced catalytic activity, which can be linked to the synergistic effect of carboxylic acid groups and unpaired electrons at the edge defects. The discovery of a simple chemical processing step to synthesize highly active graphene oxide allows the premise of industrial-scale carbocatalysis to be explored. In the drive towards green and sustainable chemistry, a constant refrain is the use of non-toxic, sustainable catalysts with minimal environmental footprint [1] , [2] , [3] . The use of carbon catalysts is attractive in this regard because of their low cost and natural abundance [4] , [5] , [6] , [7] , [8] . Carbocatalysis is well established in the oxidative dehydrogenation of ethylbenzene to produce styrene [4] . Oxidative aromatization involving a molecular oxygen and activated carbon system has also been used to prepare aromatic compounds such as pyrazoles, pyridine, indoles and so on [8] . Although the detailed mechanism of these reactions is not yet well understood, it is believed that the multiplier effect of the surface area and the dynamic exchange of oxygen functionalities in the mesopores of nanostructured carbon have important roles in promoting efficient catalysis. In this regard, graphene oxide (GO) [9] , [10] , [11] , [12] , [13] , [14] produced by the exfoliation of graphite oxide, is emerging as a versatile mediator of synthetic transformation. In many reactions, it can serve both as a supporting scaffold for various catalytically active species [15] as well as a ‘carbocatalyst’ in its own right [6] . The ability of GO to facilitate synthetic transformations stems from several intrinsic features. First, the presence of oxygen-containing functional groups allows GO to function as an oxidant for the oxidation of sulphides, [16] olefins and various hydrocarbons [17] . In addition, the acidic nature of GO allows GO to act as a solid acid for hydration, [18] Friedel–Crafts reaction, [19] Aza–Michael additions, [20] condensation [21] and ring-opening polymerization [22] . Therefore, it is attractive to develop GO-based carbocatalysts as an alternative to dwindling precious metal resources [6] , [23] . The only drawback is that the efficiency of GO is low, requiring high loading (60–400 wt%) for typical oxidative reactions [16] , [17] , [18] . In addition, the non-stoichiometric and inhomogeneous nature of GO [24] , [25] presents considerable challenges for understanding the detailed mechanism of catalysis. Here we present a detailed, systematic study to probe the catalytic activity and origin of aerobic oxidation in porous GO. Highly catalytic porous GO with enhanced catalytic activity is generated by a sequential base and an acid treatment, and yields up to 98% can be achieved with unprecedentedly low catalyst loading (5 wt %) for the oxidative coupling of amines to imines under mild conditions. Our studies suggest that carboxylic acid functionalities and spin-electrons at the edge sites are most likely involved in the aerobic oxidation of amines. Probing the catalytic activity of GO materials GO consists of both acidic and basic oxygenated groups that are solvated by water molecules. Owing to its amphiphilic nature, the chemical nature of GO sheets is influenced by the base or the acid treatments. To examine the catalytic effects of GO, several factors need to be explored. Owing to the harsh oxidation and sonication processes during its synthesis, GO sheets are usually coated by debris made of highly oxidized, and acidic molecular fragments [26] , [27] . Without a careful washing step to remove these debris, it is not clear whether the catalysis effects originate from this oxidative debris or from the intrinsic oxygen functional groups in GO. Second, contributions from metallic contaminations cannot be excluded [28] unless the GO is well purified. Therefore, as-synthesized GO sheets were subjected to the sequential base and acid treatments to eliminate acidic debris and metallic contamination ( Fig. 1 and Supplementary Fig. S1 ). 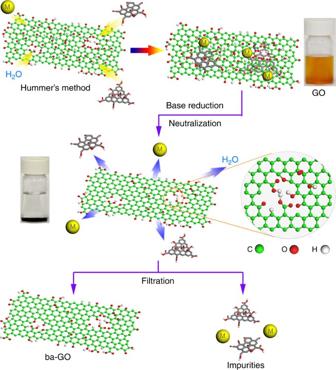Figure 1: Schematic representation of GO separation. The base reduction (NaOH, 0.1N) and acid reprotonation (HCl, 0.12 N) steps were carried out under reflux conditions to prepare modified GO (abbreviated as ba-GO), which is separated from the oxidized debris with metal (M) impurities. Figure 1: Schematic representation of GO separation. The base reduction (NaOH, 0.1N) and acid reprotonation (HCl, 0.12 N) steps were carried out under reflux conditions to prepare modified GO (abbreviated as ba-GO), which is separated from the oxidized debris with metal (M) impurities. Full size image To check whether metallic impurities were removed after the purification steps, modified GO (abbreviated as ba-GO) and its precursor graphite were analysed by inductively coupled plasma mass spectrometry ( Supplementary Table S1 ). As shown, the concentrations of all metal impurities in ba-GO are much lower than the graphite precursor and as-prepared GO. Aerobic oxidative coupling of primary amines, which often requires the use of precious metal catalyst, [29] , [30] , [31] , [32] was chosen as a model reaction, where GO and ba-GO were used as the substitute for the metal catalysts. Performing the reaction with GO and oxygen in CH 3 CN at 80 °C for 5 h results in a 44% gas chromatography (GC) yield ( Supplementary Methods ) for N -benzylidene benzylamine 2a ( Supplementary Table S2 , entry 4). Interestingly, ba-GO shows dramatically improved conversion. The optimized reaction was conducted at 80 °C with 25 mg of ba-GO and 0.5 mmol of benzylamine. The reaction was performed with continuous stirring and bubbling with oxygen for 5 h. As a result, the oxidative coupling product could be obtained with 89% GC yield ( Supplementary Table S2 , entry 8), remarkably higher than that for GO ( Supplementary Table S2 , entries 4–6). For longer times, around 6% of 2a was also converted to benzylaldehyde via hydrolysis ( Supplementary Table S2 , entry 7). Control experiments using graphite or oxidized debris recovered from the purification process produced <2% yield ( Supplementary Table S2 , entries 10–11). Control experiments were also carried out using alternative carbon catalysts similar to oxidized nanodiamond and carbon black for comparison, which all showed low activity ( Supplementary Table S2 , entries 12–13). These results prove that observed catalytic activity is unique to ba-GO, and the oxidative debris and metal contaminants do not have any significant role. In small-scale reactions, ba-GO has demonstrated its effectiveness in the oxidative coupling of various primary amines ( Supplementary Table S3 ). The applicability of this carbon catalyst has been further extended to cross-dehydrogenative coupling [33] , [34] , [35] , [36] of tetrahydroisoquinoline 3 and carbon nucleophiles 4, yielding 67–89% of coupling products 5 ( Supplementary Fig. S2 ). As GO-based materials can be readily scaled up in large quantities [37] , it is important to determine whether the scale of the catalytic process can be increased. Therefore, a 1-g scale reaction for oxidative coupling of benzylamine (9.3 mmol, 1.0 g) was investigated. We find that only 20 wt% of the catalyst loading is required for a large-scale reaction in 50 ml CH 3 CN, yielding 98% of N -benzylidene benzylamine ( Supplementary Table S2 , entry 14). We have also verified that the catalysis can be carried out in open air and similar conversion and yield can be achieved ( Supplementary Table S2 , entry 15). Performing the reaction in anaerobic conditions (glove box, oxygen<0.2 ppm) reduced the yield to 5%, thus indicating that oxygen is the terminal oxidant ( Supplementary Table S2 , entry 16). The dramatically enhanced activity of ba-GO in large-scale reaction suggests that higher concentration of substrate significantly contributes to better performance. To prove this hypothesis, we carried out the reaction under solvent-free and open-air condition, the results show that only 5 wt% of the catalyst loading is sufficient to achieve a 100% conversion with yields up to 98% ( Table 1 , entry 1). Table 1 Oxidative coupling of various primary amines catalysed by ba-GO * . Full size table With these optimized conditions, the effectiveness of ba-GO for oxidative coupling of various primary amines in a large scale was assessed ( Table 1 ). The electronic effects of the substituents on the phenyl ring are found to be well tolerated under mild reaction conditions ( Table 1 , entries 3–7). Moreover, para-, meta- and ortho-substituted benzylamine prove to be suitable substrates, revealing that the steric hindrance effect of the aryl ring has little impact on the efficiency of the coupling process ( Table 1 , entries 5–7). Catalysis of 2-thiophenemethylamine, a representative of the heterocyclic amines, can also be achieved by ba-GO with 92% yield of the corresponding product ( Table 1 , entry 8). However, when alkyl amine was subjected to the coupling reaction, much lower yield was observed by NMR, this is probably due to the inactive α -hydrogen of amine ( Table 1 , entry 9). More impressively, the ba-GO catalyst shows good recyclability and can be reused by simple filtration and rinsing in acetonitrile. There is little difference in both relative activity and selectivity ( Fig. 2 ) up to the sixth cycle tested. Above all, the performance of ba-GO is comparable or even superior to that of metal catalysts [29] , [30] , [31] . The low catalyst loading is unprecedented compared with previous catalysis reaction using GO [16] , [17] , [18] . The combination of solvent-free and metal-free catalysis using low catalyst loading is a good model for practical application. 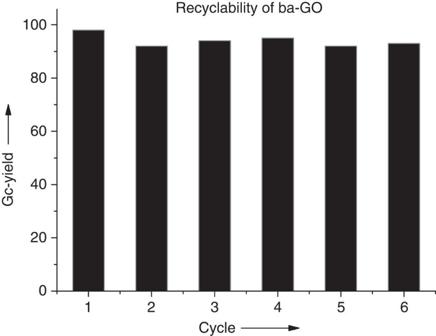Figure 2: Recyclability of ba-GO in benzylamine oxidation reaction. Conditions: 90 °C, open air, 1.0 g PhCH2NH2, 50 mg catalyst (5 wt%), 12 h. Figure 2: Recyclability of ba-GO in benzylamine oxidation reaction. Conditions: 90 °C, open air, 1.0 g PhCH 2 NH 2 , 50 mg catalyst (5 wt%), 12 h. Full size image Probing the origins of the observed catalysis It is instructive to ask this question. Why does sequential base and acid treatment (ba-GO) improve the catalytic properties of GO so significantly? (refer to Supplementary Table S2 for a comparison of the catalytic performance of ba-GO versus GO). To correlate the catalytic activity of GO with variation in its chemical structure following sequential base and acid treatments, thermal gravimetry analysis (TGA) and solid state 13 C NMR studies were performed. 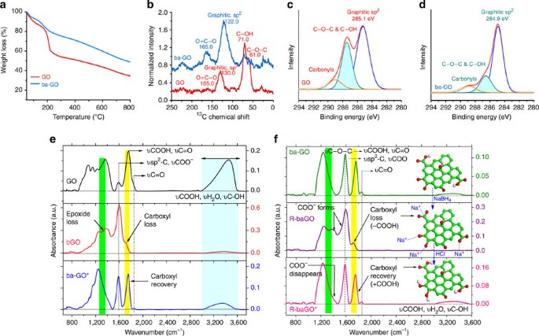Figure 3: Characterization of GO and ba-GO powder. (a) Thermal gravimetry of GO (red) and ba-GO (blue). (b)13C solid-state NMR spectra of GO (red) and ba-GO (blue). (c) X-ray photoelectron spectroscopy C1sspectra of GO and ba-GO (d). (e) Transmission infrared absorbance spectra of GO (black), b-GO (red), ba-GO* (blue) referenced to the bare substrate (cleaned oxidized silicon). (f) Transmission infrared absorbance spectra of ba-GO (green spectrum) before treating with NaBH4after treating with NaBH4at RT for 1 h (R-ba-GO, purple spectrum), followed by reprotonation by HCl at RT (R-ba-GO*, magenta spectrum). Components in the spectra due to epoxide, carboxyl and hydroxyl are highlighted in green, yellow and aqua, respectively. Figure 3a displays TGA thermograms of GO and ba-GO recorded in nitrogen atmosphere. A much lower weight loss between 150 and 300 °C is shown by the ba-GO sample compared with GO itself. This result indicates that the oxygen functional groups of ba-GO are largely removed after the base–acid treatment. 13 C NMR spectra reveal a significant decrease in the concentration of oxygen functionalities at 71.0 ppm (C-OH) and 61.9 ppm (C-O-C), which are assignable to the hydroxyl and epoxide groups. The broad resonance peak at 122.0 ppm suggests that sp 2 conjugation is partly recovered with the loss of oxygenated groups ( Fig. 3b ). X-ray photoelectron spectroscopy analysis ( Fig. 3c and Supplementary Fig. S3a ) also confirms that the populations of hydroxyl and epoxide groups become significantly reduced after stepwise base and acid treatments. According to the recent studies on the mechanism of base reduction of GO, [26] , [27] the removal of oxygen functionalities is attributed to the effective removal of oxidative fragments and to a dehydration reaction driven by the base reflux conditions [38] . Figure 3: Characterization of GO and ba-GO powder. ( a ) Thermal gravimetry of GO (red) and ba-GO (blue). ( b ) 13 C solid-state NMR spectra of GO (red) and ba-GO (blue). ( c ) X-ray photoelectron spectroscopy C1 s spectra of GO and ba-GO ( d ). ( e ) Transmission infrared absorbance spectra of GO (black), b-GO (red), ba-GO* (blue) referenced to the bare substrate (cleaned oxidized silicon). ( f ) Transmission infrared absorbance spectra of ba-GO (green spectrum) before treating with NaBH 4 after treating with NaBH 4 at RT for 1 h (R-ba-GO, purple spectrum), followed by reprotonation by HCl at RT (R-ba-GO*, magenta spectrum). Components in the spectra due to epoxide, carboxyl and hydroxyl are highlighted in green, yellow and aqua, respectively. Full size image Our purification process as well as its subsequent characterizations has excluded the role of impurities arising from debris or metallic impurities, thus the intrinsic oxygen functional groups in ba-GO should have an important role in the carbocatalysis. Fourier transform infrared (FTIR) absorption spectroscopy was performed in-situ (in a vacuum environment, see the Supplementary Methods for details) at room temperature (RT) to analyse the functional groups in base-treated GO (b-GO) and ba-GO (sequential base and acid treatments). A representative infrared absorbance spectrum of GO collected in the transmission mode is shown in Fig. 3e (black) and can be used for comparison with the spectra of b-GO, ba-GO* (b-GO followed by neutralization with the acid at RT) and ba-GO (b-GO treated with the acid at 120 °C) ( Fig. 3e ). As previously reported, [39] infrared spectra of as-synthesized GO indicate contributions from various oxygen functional groups. These groups include contributions from hydroxyls (C-OH for phenols or lactols at ~3,000–3,600 and ~1,050–1,150 cm −1 ), carbonyls (C=O, generalized for ketonic edge groups such as anhydrides, lactones and pyrones at ~1,500–1,850 cm −1 ), carboxyls (COOH at ~1650–1750, ~3,000–3,600 and ~1,050–1,200 cm −1 ), epoxides (C–O–C at ~850 and ~1,280–1,330 cm −1 ), ethers (C–O at ~800–1,200 cm −1 ) and sp 2 -hybridized C=C (sp 2 -C, in-plane vibrations at ~1,580 cm −1 ) ( Fig. 3e , black). In contrast to GO, the intensity of the hydroxyl band at ~3,000–3,600 cm −1 in b-GO ( Fig. 3e , red) is low. The carboxyl band at ~1,650–1,750 cm −1 is also considerably weaker, whereas the sp 2 -C mode at ~1,580 cm −1 is stronger. This spectral information suggests an increase of sp 2 -conjugated domain density in the carbon backbone following the base treatment, which overlaps with the possible contributions from carboxylates (COO − ). The bands at ~1,750–1,800 cm −1 originate from ketones or quinones as these are stable in basic conditions [39] . To find out whether the functional groups that are affected by the base treatment can be regenerated, b-GO was immersed in a HCl solution (0.1M) at RT for 1 h to produce ba-GO*. Following such a treatment, intensity of the carboxyl peak (~1,650–1,750 and ~1,050–1,200 cm −1 ) increases, due to the reprotonation of COO – groups. This observation also confirms the presence of such carboxyl groups after the base treatment. However, hydroxyls (~3,000–3,600 and ~1,050–1,150 cm −1 ) and epoxides (~850 and ~1,280–1,330 cm −1 ) could not be recovered ( Fig. 3e , blue). Spectral analysis of both ba-GO* and thermally treated GO ( Supplementary Fig. S4 ) further revealed the fact that the base treatment produced similar effect as thermal treatment in chemically reducing the hydroxyl and epoxy species. In both of these processes, the intensity of sp 2 -conjugated C=C stretch ~1,580 cm −1 recovered as shown in Supplementary Fig. S5 . The differences in the intensity of the hydroxyl bands between ba-GO* (b-GO treated with the acid at RT) and ba-GO (b-GO treated with the acid at a high temperatures) suggest that hydroxyl groups (~3,000–3,600 and ~1,050–1,150 cm −1 ) could be further removed during the acid-refluxing process ( Fig. 3e , blue and Fig. 3f , green). After sequential base and acid treatments, in-situ FTIR analysis reveals that the residual oxygen functional groups in ba-GO are mainly ketones, epoxides (significantly reduced) and carboxylic acids. The hydroxyl groups have been largely removed. To test how the catalysis is affected by the further reduction of residual oxygen functional groups, ba-GO were treated with NaBH 4 ( Fig. 3f , purple), a well-known reducing agent for GO [12] . Indeed, the yield was reduced dramatically to 11% in the oxidative coupling of benzylamine ( Supplementary Table S2 , entry 18). However, reduction in the catalytic efficiency can either originate from the reduction of the oxygen-functionalities such as quinones, epoxides or from the deprotonation of the carboxylic acid groups. To investigate whether the base effect of NaBH 4 has affected the catalytic reaction, a neutralization step with acid ( Fig. 3f , magenta) was carried out at RT. This resulted in a regeneration of the carboxyl peak at ~1,650–1,750 cm −1 along with a remarkable recovery of the catalytic activity with a 78% yield ( Supplementary Table S2 , entry 19). This finding therefore provides strong evidence that the carboxylic acid groups have a vital role in the catalysis reactions as it is unlikely that the neutralization treatment can recover the reduced oxygen functionalities or introduce additional oxygen functionalities. This explanation agrees well with our observation that the catalytic properties of base-treated GO (b-GO) is much poorer than those of the ba-GO and the catalytic activity is enhanced only after the acid neutralization ( Supplementary Table S2 , entries 8 and 20). All these findings point strongly to the significant contribution of the carboxylic acids in the catalytic conversion here. To confirm the role of carboxylic acids in this synthetic transformation, 1-pyrene carboxylic acid was used as a molecular analogue to mimic the graphene-based catalytic system. To our delight, 1-pyrenecarboxylic acid exhibits a 95% yield in the oxidative coupling of benzylamine ( Supplementary Table S4 , entry 2), which is comparable with the activity of ba-GO. We also observed that pyrene itself has no activity in the aerobic oxidation of amines. We have further tested a large range of carboxylic acids without large π-conjugation system, and these did not exhibit any reactivity ( Supplementary Table S4 ). According to the widely accepted Lerf–Klinowski model, [40] epoxy and hydroxyl groups reside on the GO basal plane, whereas the periphery of the GO sheets is decorated mainly by carboxyl, anhydride, lactone, phenol, lactol or pyrone groups. As the carboxylic acids are mainly residing at the periphery of the sheet, its coverage will be expected to be relatively low compared with the other oxygenated groups and it is difficult to explain the observed catalytic activity. Scanning tunnelling microscope (STM) imaging ( Fig. 4 ) reveals that GO sheets become highly porous after the base treatment with an average pore area of around 5 nm 2 . These holes could be created during the harsh oxidation process, which were enlarged by the etching process during the base treatment. Infrared spectroscopy studies also confirmed the hole defect formation by indicating a CO 2 production during thermal annealing of base-treated GO ( Supplementary Fig. S6 ). This fact could be further confirmed by atomic force microscopy studies ( Supplementary Fig. S7 ). These findings suggested that the active catalysis sites in ba-GO are likely to be hole defects in the conjugated domain, and the edges of the hole defect are terminated by the carboxylic acids. 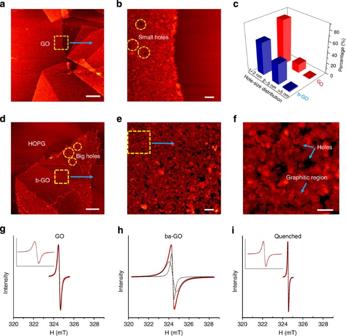Figure 4: STM and ESR measurement of GO materials before and after chemical treatment. (a) STM images of GO after annealing at 375 K for 10 mins (1 × 1 μm). A low temperature annealing is needed to remove adsorbates to allow clear imaging. (b) Magnified views of GO sheet (100 × 100 nm). (c) Histogram of hole size distribution. The density of larger-sized holes is higher in b-GO relative to GO. (d) STM images of b-GO: after annealing at 375 K for 10 min. (e) Magnified views of b-GO, 100 × 100 nm. (f) Magnified views of b-GO, 26 × 26 nm. (g) ESR spectra for GO, ba-GO (h) and ba-GO-PhCOOH (i). The solid lines are fitted with Lorentzian curves. The magnified spectra for GO and ba-GO-PhCOOH are shown in the inset. The scale bars, 100 nm (a,d), 10 nm (b,e) and 4 nm (f). Figure 4: STM and ESR measurement of GO materials before and after chemical treatment. ( a ) STM images of GO after annealing at 375 K for 10 mins (1 × 1 μm). A low temperature annealing is needed to remove adsorbates to allow clear imaging. ( b ) Magnified views of GO sheet (100 × 100 nm). ( c ) Histogram of hole size distribution. The density of larger-sized holes is higher in b-GO relative to GO. ( d ) STM images of b-GO: after annealing at 375 K for 10 min. ( e ) Magnified views of b-GO, 100 × 100 nm. ( f ) Magnified views of b-GO, 26 × 26 nm. ( g ) ESR spectra for GO, ba-GO ( h ) and ba-GO-PhCOOH ( i ). The solid lines are fitted with Lorentzian curves. The magnified spectra for GO and ba-GO-PhCOOH are shown in the inset. The scale bars, 100 nm ( a , d ), 10 nm ( b , e ) and 4 nm ( f ). Full size image Our studies showed that the base reduction of GO generates nanovoids that are surrounded by conjugated domains. Localized spins originating from the non-bonding π electron states are likely to be created at the edges, analogous to non-kekulè molecules having open shell unpaired electrons. To confirm this fact, we performed electron spin resonance (ESR) measurements for GO subjected to different treatments. The ESR spectra shown in Fig. 4g–i can be fitted by two kinds of Lorentzian curves; one having a narrower linewidth and the other with a broader one. Sharper peaks appear in all samples, with linewidth close to that for sigma dangling bond spins observed in nanoporous carbon materials (~0.1 mT) [41] . On the other hand, the broader peak, which is only observed in ba-GO, has a linewidth similar to that of localized spins originating from the edge of nanographene (~1 mT) [42] , [43] . The π-electron radical at the edges of graphene is delocalized along the edges to some extent, and exhibits fast spin-lattice relaxation through interaction with the adjacent π-electron system, giving rise to a broad linewidth in ESR. Only ba-GO exhibits the broader ESR signal, with an intensity ratio of the broad peak to narrow peak of about 5:1. Therefore, it can be inferred that the observed catalytic ability is related to the localized spins created at the edge of π-electron system. One way to study whether the spin states are important in catalysis is to quench them. It is well known that the coupling of diazonium to graphene occurs via a radical pathway, and therefore regions on graphene with unpaired electrons should be highly reactive towards such coupling reactions. In this case, we functionalized ba-GO with phenyl carboxylic acid using diazonium coupling reactions. Introduction of the phenyl carboxylic groups ensures that the density of the carboxylic functionalities is preserved after the coupling reactions, although the density of unpaired spins in ba-GO will be reduced. Indeed, the ESR response of the broad peak is now significantly reduced after the diazonium coupling, and this is associated with the decrease in the catalytic activity of ba-GO-PhCOOH from 89 to 30% in the oxidative coupling of benzylamine ( Supplementary Table S2 , entries 8 and 21). This suggests that radical states at the edge sites are important in the catalysis besides carboxylic groups. To shed light on the mechanism, we employed a spin-trapping electron paramagnetic resonance (EPR) technique using 5,5-dimethyl-1-pyrroline N -oxide (DMPO) as the spin trap to detect the intermediates formed during reaction. DMPO is a particularly useful probe for trapping oxygen-derived radicals (for example, ·O 2 − radicals) because of the relative stability and the diverse spectral characteristics of the spin adducts. As shown below, the EPR signal shows the characteristic fingerprint of spin adducts due to superoxide radical (·O 2 − ) (DMPO·OO(H)). Control studies show that in the absence of ba-GO catalyst or O 2 , spin signals due to oxygen radical show very low intensity ( Fig. 5b ). The formation of H 2 O 2 , which is one of the postulated intermediates in the aerobic oxidation reactions is also detected by using the catalysed oxidation of N , N -diethyl-1, 4-phenylenediammonium sulphate (DPD) by Horseradish peroxidase (POD), where two absorption peaks centred at ca. 510 and 551 nm ( Fig. 5c ) can be seen. These result show that the aerobic oxidation in our catalytic system proceeds via superoxide radical (·O 2 − ) and H 2 O 2 is the intermediate product. 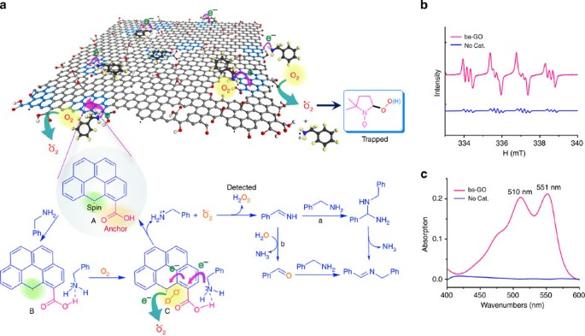Figure 5: Mechanism of ba-GO catalysed oxidative coupling of primary amines. (a) Schematic representation of the oxidation mechanism. (b) The DMPO spin-trapped EPR spectra with or without catalyst; in the presence of ba-GO catalyst and O2, spin signals due to DMPO-OO(H) show much higher intensity and are the predominant signals. (c) The ultraviolet-visible absorption spectra of reaction system with or without catalyst after adding DPD and POD. Figure 5: Mechanism of ba-GO catalysed oxidative coupling of primary amines. ( a ) Schematic representation of the oxidation mechanism. ( b ) The DMPO spin-trapped EPR spectra with or without catalyst; in the presence of ba-GO catalyst and O 2 , spin signals due to DMPO-OO(H) show much higher intensity and are the predominant signals. ( c ) The ultraviolet-visible absorption spectra of reaction system with or without catalyst after adding DPD and POD. Full size image We suggest that these edge sites with unpaired electrons constitute the active catalytic sites and afford enhanced kinetics for the trapping and activation of molecular oxygen by a sequence of electron transport and reduction to superoxide radical. One plausible mechanism involving both the unpaired electron and the carboxylic groups is proposed as following: Benzylamine 1a binds to the acidic carboxyl groups via hydrogen bond, and forms an electron-donor complex B . The unpaired electrons of porous GO reduce molecular oxygen to form ·O 2 − , which stays surface-bound to the GO to stabilize the positive charge of the hole. At the same time, the anchored amine is oxidized by positive charge of the hole to form the cation radical complex. The superoxide radical (·O 2 − ) can abstract hydrogen atom from the amine radial cation to produce imine intermediates and H 2 O 2 . Meanwhile, the active site is released for another catalytic cycle, giving rise to a turnover mechanism. The imine intermediates can react with the free amines to furnish the coupling products ( Fig. 5a , pathway a) or with water to produce benzaldehydes, which are then transferred to coupling products via condensation reactions shown with 1a ( Fig. 5a , pathway b). The role of base and acid treatment in enhancing the catalytic performance of GO can now be understood. Refluxing in base helps to increase the density of the nanovoids in GO, which gives rise to a high density of edges that can have localized spins. Another important effect of the base reduction is the removal of the hydroxyl groups. This has the effect of changing the dynamics of water solvation layer around GO, which allows greater access to the catalytic sites by the reactant. A subsequent acid neutralization step is needed to recover the active carboxylic groups, which serves as hydrogen bonding sites to the amines and also facilitates the proton transfer reactions due to its acidic properties. More excitingly, we discovered that ba-GO catalyst can be used under solvent-free, open-air condition and is recyclable, this has tremendous implication for green catalysis and the full potential of this material remains to be discovered. In conclusion, we have identified a chemical treatment that is needed to impart high catalytic activities on GO in the aerobic oxidation of various amines and investigated the catalytic origins. As GO is an amphiphilic material with pH-sensitive functional groups, appropriate base and acid treatments are needed to activate the catalytic sites in GO. The carboxylic groups at the edges of defects, along with the localized unpaired electrons, work synergistically to trap molecular oxygen and the amine molecules, thus facilitating intermolecular arrangements. In view of the fact that the production of GO is now being scaled up industrially, these chemical processing steps can be adopted as the standard protocol to render GO catalytically active, thus opening the possibility for the large-scale industrial applications of GO in industrial catalysis. Base–acid treatment of graphene oxide (ba-GO) The as-produced GO was dispersed in 750 ml DI water at a concentration of 0.6 mg ml −1 . Three grams of NaOH plate was added into GO solution (0.1 mol l −1 ). The mixture was refluxed in a round-bottom flask under constant magnetic stirring for 1 h. Subsequently, the base-treated GO were separated by centrifuging at 13,000 r.p.m. and dispersing in 750 ml DI water. Then, 7.5 ml HCl (37%) was added into the solution slowly. The mixture was refluxed for another 1 h. The final ba-GO obtained were filtered and washed by DI water and acetone. The synthesized ba-GO was kept in vacuum desiccators. Debris ( Supplementary Fig. S7a and Supplementary Fig. S8 ) present in the GO solution was isolated by using ammonia as the base according to the reported reference [26] . Synthesis of compound 2a in CH 3 CN The obtained ba-GO (200 mg) was dispersed in acetonitrile (50 ml) in round-bottom flask and ultrasonicated for 1 h. Benzylamine (1.0 g) was added into the solution. The mixture was stirred with continual oxygen bubbling and slightly refluxed for 10 h. After that, the solution was cooled to RT and 1.0 g of anisole was added. The reaction mixture samples were taken out by syringe and checked by GC–MS: 98% GC Yield. ba-GO catalyst can be recovered by simple filtration and rising in CH 3 CN ( Supplementary Fig. S9 ). Solvent-free and aerobic synthesis of compound 2a The obtained ba-GO (50 mg) was dispersed in 1.0 g of benzylamine and ultrasonicated for 30 min. The mixture was stirred at 90 °C for 12 h under open air. After that, the solution was cooled to RT and 1.0 g of anisole was added. After filtration and washing by CH 3 CN, aliquots of the mixture were extracted using a syringe and checked by GC–MS (98% GC-yield). Evaporation under vacuum (2 mbar, 65 °C) afforded 2a in 95% yield (867 mg). 1 H NMR (300 MHz, CDCl 3 , 25 °C, TMS): δ =8.45 (s, 1H), 7.80−8.00 (m, 2H), 7.20−7.60 (m, 8H), 4.89 ppm (s, 2H); 13 C NMR (75 MHz, CDCl 3 , 25 °C, TMS): δ =65.0, 126.9, 127.9, 128.2, 128.4, 128.5, 130.7, 136.1, 139.2, 161.9 ppm; MS (70 eV, EI) m/z : 195 (M + ). ba-GO catalyst can be reused for multi-runs by simple filtration and rising in CH 3 CN. Synthesis of compound 5a The as-made ba-GO (40 mg) was dispersed in acetonitrile (10 ml) in a round-bottom flask and ultrasonicated for 1 h. N -phenyl tetrahydroisoquinoline 3a (52.3 mg) and nitromethane (0.2 ml) was added into the solution. The mixture was stirred with continual oxygen bubbling and slightly refluxed for 24 h. Filtration, evaporation and column chromatography on silica gel afforded 5a in 78% yield (52.0 mg). 1 H NMR (300 MHz, CDCl 3 , 25 °C, TMS): δ =7.16−7.40 (m, 6H), 7.03 (d, J =7.9 Hz, 2H), 6.90 (t, J =7.3 Hz, 1H), 5.60 (t, J =7.2 Hz, 1H), 4.92 (dd, J1 =7.7 Hz, J2 =11.8 Hz, 1H), 4.92 (dd, J1 =6.6 Hz, J2 =11.9 Hz, 1H), 3.60−3.80 (m, 2H), 3.06−3.20 (m, 1H), 2.76−2.90 ppm (m, 1H); 13 C NMR (75 MHz, CDCl 3 , 25 °C, TMS): δ =26.4, 42.0, 58.1, 78.7, 115.1, 119.4, 126.6, 126.9, 128.1, 129.1, 129.4, 132.9, 135.2, 148.4 ppm. ESR measurements for GO samples ESR measurements were performed with an ESR X-band spectrometer (JEOL JES-TE200) at RT for typically 4.5 mg samples sealed in a quartz sample tube. The samples were evacuated to <10 −6 Torr at RT for 20 h to avoid influence of adsorbed oxygen, which often bury the intrinsic ESR signals of porous material in advance. The incident microwave power of 250 μW, where saturation does not occur, is applied for excitation. Detecting H 2 O 2 Sample preparation: DPD reagent was prepared by dissolving 0.1 g of DPD in 10 ml 0.05 mol l −1 H 2 SO 4 and stored in dark at 5 °C. POD reagent was prepared by dissolving l0 mg peroxidase product from horseradish in 10 ml of tridistilled water. The standard solution was stored at 5 °C. Both DPD and POD were prepared freshly on demand. Typical procedure for the detection of H 2 O 2 : The obtained ba-GO (25 mg) was dispersed in CH 3 CN (10 ml) and ultrasonicated for 1 h. Benzylamine (53.5 mg, 0.5 mmol) was added into the solution. The mixture was stirred at 80 °C for 5 h. After that, the solution was cooled to RT and filtered to remove ba-GO. Twenty milliliter DI water was added to the solution, and the mixture was further extracted by EtOAc (20 ml × 3) to remove the organic compounds. The aqueous solution was diluted to 400 ml by DI water. 9 ml aqueous solution and 1 ml PBS buffer (pH 7.4) was added into the beaker with stirring, and used as the test sample. The ultraviolet-visible spectra of test sample were recorded after adding 20 μl DPD and 20 μl POD. The mixture that contains all reagents except POD was used to record the baseline absorption ( Supplementary Fig. S10 ). Detecting superoxide radical anion Typical spectrometer parameters: Microwave power: 20 mW. Microwave Freq. : 9.4 GHz. Scan time: 1 min. Modulation amplitude: 0.02 mT. Modulation Freq.:100 kHz. Receiver gain: 10 × 2. Time constant: 0.01. Typical EPR spectra of reaction system: ba-GO (25 mg), Benzylamine 1a (53.5 mg, 0.5 mmol), MeOH (2 ml). The reaction mixture was vigorously stirred at 60 °C bubbling with oxygen for 0.5 h. This reaction solution was taken out into a small tube followed by the addition of DMPO. Then, the mixture was analysed by EPR ( Supplementary Fig. S11 ). Characterization SEM images were recorded using the JEOL 6701 FESEM (field emission scanning electron microscopy) at 30 kV. STM images were recorded in the constant current mode at RT after annealing the samples at specified temperature. Atomic force microscopy images were collected using the X100c, and the specimens studied were coated freshly on highly ordered pyrolytic graphite (HOPG) substrates by spin coating. TGA and differential thermal analysis were recorded using a Rigaku TG8101D and TAS 300 data-processing system with an aluminium pan under N 2 with a heating rate of 10 °C min −1 . X-ray photoelectron spectroscopy was performed with the Phobios 100 electron analyzer equipped with 5 channeltrons, using an unmonochromated Al Kα X-ray source (1,486.6 eV). ESR measurements were performed with an ESR X-band spectrometer (JEOL JES-TE200) at RT for typically 4.5 mg samples sealed in a quartz sample tube. FTIR measurements were performed at RT in a continuous vacuum environment with data collected typically 500 scans per loop in the transmission mode. A deuterated triglycine sulphate detector having a mirror optical velocity of 0.6329, cm s −1 was used at a 4 cm −1 resolution. The samples were placed in an annealing chamber and positioned at an infrared incident angle close to the Brewster’s angle (70°). For annealing studies, data collection per loop was performed at 60 °C. The annealing time was 5 mins at each temperature for a stepwise reduction and the total annealing time for the overall experiment per sample was ~8 h. See more details in Supplementary Methods section. How to cite this article: Su, C. et al . Probing the catalytic activity of porous graphene oxide and the origin of this behaviour. Nat. Commun . 3:1298 doi: 10.1038/ncomms2315 (2012).